High-capacity millimetre-wave communications with orbital angular momentum multiplexing One property of electromagnetic waves that has been recently explored is the ability to multiplex multiple beams, such that each beam has a unique helical phase front. The amount of phase front ‘twisting’ indicates the orbital angular momentum state number, and beams with different orbital angular momentum are orthogonal. Such orbital angular momentum based multiplexing can potentially increase the system capacity and spectral efficiency of millimetre-wave wireless communication links with a single aperture pair by transmitting multiple coaxial data streams. Here we demonstrate a 32-Gbit s −1 millimetre-wave link over 2.5 metres with a spectral efficiency of ~16 bit s −1 Hz −1 using four independent orbital–angular momentum beams on each of two polarizations. All eight orbital angular momentum channels are recovered with bit-error rates below 3.8 × 10 −3 . In addition, we demonstrate a millimetre-wave orbital angular momentum mode demultiplexer to demultiplex four orbital angular momentum channels with crosstalk less than −12.5 dB and show an 8-Gbit s −1 link containing two orbital angular momentum beams on each of two polarizations. Although electromagnetic (EM) waves have been studied for well over a century, one property of EM waves, namely orbital angular momentum (OAM), was discovered in the 1990s. This discovery, along with the studies that followed, promised to enable the transmission of many independent data streams over the same spatial wireless medium [1] , [2] . An EM wave carrying OAM has a helical transverse phase structure of exp ( iℓφ ), in which φ is the transverse azimuthal angle and ℓ is an unbounded integer (the OAM state number). Note that OAM relates to the spatial phase profile rather than to the state of polarization of the beam, which is associated with spin angular momentum [3] . OAM beams with different ℓ values are mutually orthogonal, allowing them to be multiplexed together along the same beam axis and demultiplexed with low crosstalk [2] , [4] , [5] . Consequently, one can establish a well-defined line-of-sight link for which each OAM beam at the same carrier frequency can carry an independent data stream, thereby increasing the capacity and spectral efficiency by a factor equal to the number of OAM states. Indeed, OAM has seen exciting progress in the optical domain. Systems results have shown Tbit s −1 transmission over both free-space and special vortex fibre, in which all OAM beams are multiplexed together and propagate along the same spatial axis [6] , [7] . Importantly, given that the demand for capacity and spectral efficiency continues growing exponentially because of the multitude of wireless applications, including data centre and back-haul connections [8] , [9] , [10] , [11] , [12] , there is great interest to also show advanced multiplexing approaches at radio frequency (RF) and millimetre-wave (mm-wave) frequencies. However, given the different frequency range from optics, such RF and mm-wave systems would require different technologies to achieve the desired results. Specifically, RF and mm-waves transmitted and received using a single aperture pair (that is, the data pass through one aperture at the transmitter and are received by another aperture at the receiver) have been used for free-space wireless communications since the days of Marconi [13] , [14] , [15] . Although there have been many advances since that time, such as advanced modulation format and polarization multiplexing, the basic system architecture has remained fairly unchanged. Thus, OAM mode multiplexing of multiple orthogonal data-carrying beams multiplexed at the transmitter and demultiplexed at the receiver using a single transmitter/receiver aperture pair would represent a significant architectural change. Recent reports have shown that OAM beams can be used for data transmission in RF links [16] , [17] , including the transmission of one Gaussian and two OAM beams ( ℓ= 0, ±1), each carrying an 11-Mbit s −1 signal at an ~17-GHz carrier frequency [18] , [19] , [20] . However, different OAM beams in these demonstrations propagate along different spatial axes and are not transmitted through the same aperture. Note that coaxially propagating OAM beams could enable certain advantages, such as (a) inherently low crosstalk among OAM channels, (b) reduced need for further signal processing to cancel OAM channel interference after demultiplexing and (c) scalability to increase the number of OAM channels [6] . In order to fully exploit the advantages of OAM mode-division multiplexing, OAM channels should be multiplexed and transmitted along the same spatial axis though a single aperture. In this article, we demonstrate a high-capacity mm-wave communication link by transmitting eight multiplexed OAM beams (four OAM beams on each of the two orthogonal polarizations), each carrying a 4 × 1 Gbit s −1 (4 bits per symbol) quadrature amplitude modulation (16-QAM) signal, thereby achieving a capacity of 32 Gbit s −1 (1 Gbaud × 4 bit per symbol × 4 OAM beams × 2 polarizations) and a spectral efficiency of ~16 bit s −1 Hz −1 at a single carrier frequency of 28 GHz (ref. 21 ). Four OAM beams with state numbers −3, −1, +1 and +3 on each of two polarizations are generated and multiplexed using spiral phase plates (SPPs) made out of high-density polyethylene (HDPE) and specially designed beamsplitters (BSs) at the transmitter, such that all beams co-propagate from a single transmitter aperture. After propagating through 2.5 m, the OAM channels are demultiplexed at the receiver using two techniques: (a) SPPs [22] , which can convert an OAM beam back into an approximate Gaussian beam and (b) a mm-wave OAM mode demultiplexer for demultiplexing multiple OAM beams. The on-axis propagation of all OAM channels and the orthogonality among them allow their demultiplexing to be accomplished using physical microwave components with low crosstalk, reducing the need for further signal processing to cancel channel interference [23] . 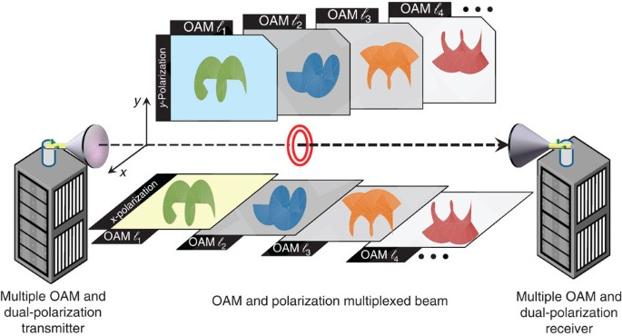Figure 1: Concept of utilizing OAM and polarization multiplexing in a free-space mm-wave communication link. This technique could have potential applications in places, such as data centres, where large bandwidth links between computer clusters are required. Generation and multiplexing of eight mm-wave OAM channels Figure 1 illustrates a prospective application scenario of using OAM multiplexing for short range, high-speed wireless information exchange in a data centre. In this paper, we demonstrate a proof-of-concept experiment under laboratory conditions. A schematic overview of an OAM-multiplexed mm-wave communication link is shown in Fig. 2a . We generate each mm-wave OAM beam of state ℓ by passing polarization-multiplexed (pol-muxed) Gaussian beams, emitted by a collimated dual-polarization, lensed-horn antenna, through an SPP (see Fig. 2b ). In general, mm-wave OAM beams can be generated using different techniques (for example, holographic plates [17] and SPPs [22] ). In our system, we choose to use SPPs made out of HDPE for convenience because of our in-house machining capability. The SPP is defined by its thickness, which varies azimuthally according to , acquiring a maximum thickness difference of Δ h = ℓλ/(n −1) ( φ is the azimuthal angle varying from 0 to 2π , n is the refractive index of the plate material and λ is the wavelength of the mm-wave) [4] . Normally, one surface of an SPP is flat; therefore, the required thickness can be obtained simply by controlling the height of the other surface. These SPPs are manufactured through the computer numerical control milling of a solid block of HDPE, which has a refractive index of n =1.52 at 28 GHz. The SPPs that are used to generate the OAM beams have circular apertures with diameters of 30 cm. The size of the SPP is larger than that of the lensed-horn antenna in order to limit possible effects that may arise from a truncated aperture. We note that the SPP is placed after the antenna such that the Gaussian beam diameter is smaller than the diameter of the SPP. For the four OAM states used in this experiment, the SPPs corresponding to ℓ =±1 and ℓ =±3 are designed to have height differences of Δ h 1 =±2.07 cm and Δ h 3 =±6.21 cm, respectively (see Supplementary Fig. 1 and Supplementary Note 1 ). Figure 1: Concept of utilizing OAM and polarization multiplexing in a free-space mm-wave communication link. This technique could have potential applications in places, such as data centres, where large bandwidth links between computer clusters are required. 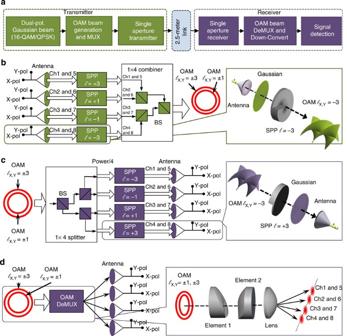Figure 2: Experiment of OAM and polarization multiplexing in a free-space mm-wave communication link. (a) Schematic diagram of a millimetre-wave link based on OAM and polarization multiplexing. (b) Polarization-multiplexed (pol-muxed) OAM beams (ℓ=−3, −1, +1 and +3) are generated by dual-polarization lensed-horn antennae, followed by SPPs. These beams are multiplexed by a 1 × 4 combiner (three beamsplitters in our experiment). (c) SPP-based OAM demultiplexer. The received OAM beams are split into four copies by a 1 × 4 splitter (three beamsplitters), for each of which (ℓ) is demultiplexed and converted into a Gaussian beam by a reverse SPP of (−ℓ). (d) OAM mode demultiplexer. The received OAM beams are demultiplexed by an OAM mode demultiplexer, which can spatially separate the four OAM beams without power-splitting loss. Pol: polarization, MUX: multiplexing, DeMUX: demultiplexing, Ch: channel, BS: beamsplitter. Full size image Figure 2: Experiment of OAM and polarization multiplexing in a free-space mm-wave communication link. ( a ) Schematic diagram of a millimetre-wave link based on OAM and polarization multiplexing. ( b ) Polarization-multiplexed (pol-muxed) OAM beams ( ℓ =−3, −1, +1 and +3) are generated by dual-polarization lensed-horn antennae, followed by SPPs. These beams are multiplexed by a 1 × 4 combiner (three beamsplitters in our experiment). ( c ) SPP-based OAM demultiplexer. The received OAM beams are split into four copies by a 1 × 4 splitter (three beamsplitters), for each of which ( ℓ ) is demultiplexed and converted into a Gaussian beam by a reverse SPP of (− ℓ ). ( d ) OAM mode demultiplexer. The received OAM beams are demultiplexed by an OAM mode demultiplexer, which can spatially separate the four OAM beams without power-splitting loss. Pol: polarization, MUX: multiplexing, DeMUX: demultiplexing, Ch: channel, BS: beamsplitter. Full size image To verify the characteristics of the generated OAM beams, their spatial normalized intensity and interferogram are captured via a probe antenna with a small aperture diameter of 0.7 cm. The output of this antenna is recorded by an RF spectrum analyser. The probe antenna is attached to a two-dimensional (2D) linear translation stage with a scanning resolution of 1 cm and a transversal coverage area of 60 × 60 cm. 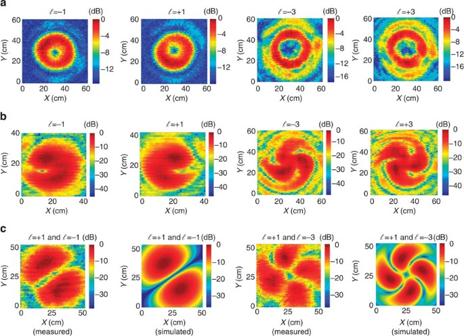Figure 3: Normalized intensity and interferogram of mm-wave OAM beams. (a) Normalized measured intensity of four mm-wave OAM beams of chargeℓ=±1 andℓ=±3. (b) Interferogram images of a Gaussian beam and OAM beams combined by a beam splitter. (c) Normalized measured and simulated intensity distribution of the multiplexed OAM beams after beam splitters. Figure 3a clearly depicts the ring-shaped normalized intensity profile [24] of the generated OAM beams. The state number of the OAM beams can be deduced from the number of rotating arms in their interferograms, as shown in Fig. 3b , which are generated by interfering the different OAM beams with a Gaussian beam ( ℓ =0) using a BS, as described below. The field distribution of an SPP-generated OAM beam created via a fundamental Gaussian beam is similar to a Laguerre–Gaussian (LG) mode [1] . The OAM state of such a beam is preserved as it propagates in free space. One can consider that such an SPP-generated OAM beam is a superposition of multiple LG modes, each with the same azimuthal index ℓ but with a different radial index p (refs 4 , 22 ). Figure 3c shows the normalized measured intensity distributions of the coherent superposition of different OAM beams, which are in good agreement with the corresponding simulation results. Figure 3: Normalized intensity and interferogram of mm-wave OAM beams. ( a ) Normalized measured intensity of four mm-wave OAM beams of charge ℓ =±1 and ℓ =±3. ( b ) Interferogram images of a Gaussian beam and OAM beams combined by a beam splitter. ( c ) Normalized measured and simulated intensity distribution of the multiplexed OAM beams after beam splitters. Full size image Eight pol-muxed OAM beams generated by four dual-pol lensed-horn antennae, each followed by an SPP with a different ℓ value, are spatially multiplexed via a 1 × 4 combiner (comprising three cascaded 50:50 planar BSs, as shown in Fig. 2b ). Our BSs are similar in form to the polka-dot BSs used in the optical regime. These BSs are implemented by spatially varying the reflectivity of the surface. This is achieved by designing an array of reflective material on a dielectric substrate to obtain 50% transmission and 50% reflection at a frequency of 28 GHz. In our experiment, the BSs are fabricated by patterning a standard printed circuit board with the designed structure (see Supplementary Fig. 2 and Supplementary Note 2 ). The eight multiplexed OAM channels (four OAM states on each of two orthogonal polarizations) are obtained by combining OAM beams of ℓ= ±1 and ℓ= ±3 using a 1 × 4 beam combiner. The divergence of the OAM beams is related to the OAM state number ℓ . For example, the sizes of propagating LG beams are proportional to the square root of | ℓ |, given that they have the same Rayleigh range [25] . To resolve this ℓ -dependent divergence, convex RF lenses made of HDPE with focal lengths of 2 m are fabricated and used to slightly focus the ℓ= ±3 modes so that their beam sizes become similar to that of the OAM beams of ℓ= ±1 at the receiver over the designed link length of 2.5 m. The resulting eight coaxial channels, each carrying an independent 1-Gbaud 16-QAM data stream, co-propagate towards the receiver, transmitting a total of 32-Gbit s −1 on a single RF carrier of 28 GHz (See Supplementary Fig. 3 and Supplementary Note 3 for the generation of a 1-Gbaud 16-QAM signal). Link capacity measurement of eight multiplexed OAM channels In the experiment using the SPP-based receiver, we recover eight multiplexed OAM channels one at a time by using a corresponding SPP and an antenna [26] . To recover an OAM beam ( ℓ ) of interest, an inverse SPP with a specific state (− ℓ ) is used to remove the azimuthal phase term exp ( iℓφ ) of the OAM beam, which is then converted back into a beam with a planar phase front of ℓ= 0. This beam then has a bright high-intensity spot at the centre, which is separable from OAM beams with ‘doughnut’ intensity profiles through spatial filtering. For example, in order to obtain the pol-muxed data streams of the ℓ=−3 OAM beam (created by an SPP with a thickness profile of ), an inverse SPP with the opposite thickness profile of is employed (see Fig. 2c ). Note that the transmitter and receiver lensed-horn antennae are matched to the Gaussian beams ( ℓ =0). Consequently, the helical phase of the ℓ =−3 OAM beam is removed, and the emerging wave can be collected with a dual-polarization lensed-horn antenna. All other beams, while also transformed by the SPP ( ℓ= +1→ ℓ =+4, ℓ= −1→ ℓ =+2 and ℓ= +3→ ℓ =+6), maintain their ring-shaped profiles and helical phase, and therefore, negligible signals can be coupled into the Gaussian-matched antenna because of the mode mismatch. Our measurements do not show an appreciable sensitivity to the rotation of the SPP at the receiver. We believe that this is because of the helical structure of the SPP. The output from this dual-polarization receiver antenna is recorded and digitized with an 80-Gsample s −1 real-time oscilloscope with an analogue bandwidth of 32 GHz, which is wide enough to faithfully capture the modulated 28 GHz mm-wave waveforms. The recorded signals are then processed offline to recover the 16-QAM constellations and calculate the bit-error rate (BER; See Supplementary Note 4 for the detection of a 1-Gbaud 16-QAM signal). The transmitted signal power and link budget are characterized as follows. The generated signal power of 8 dBm is fed into the lensed-horn transmitter antenna. The baseline power loss of the link, including the two lensed-horn antennae but excluding the SPPs, is ~22 dB. The power loss of the link increases to ~33 dB once two SPPs are inserted for OAM generation and back conversion. Furthermore, each OAM beam passes through two BSs for multiplexing at the transmitter, resulting in an additional ~6-dB power loss. Therefore, the total power loss for the link is ~39 dB. It is expected that the power from other channels would leak into the channel under detection because of the imperfections of OAM generation, multiplexing and set-up misalignment, which would essentially result in channel crosstalk when a specific channel is recovered at the receiver. The crosstalk for a specific OAM channel ℓ 1 can be measured by , where is the received power of channel ℓ 1 when all channels except channel ℓ 1 are transmitted, and is the received power of channel ℓ 1 when only channel ℓ 1 is transmitted. Given that our RF-modulated signal spectrally lies within 28±1 GHz and the fact that our SPPs and BSs are frequency-dependent, for the sake of simplification, we only measure the crosstalk at the frequencies of 27.5, 28 and 28.5 GHz for each channel by transmitting a continuous wave (CW) signal rather than 1-Gbaud 16-QAM -modulated signals. For example, to obtain the crosstalk for channel ℓ =−1, we measure the total received power from channels ℓ =+1, ±3 and divide it by the received power from channel ℓ =−1. Table 1 presents the crosstalk of each OAM channel measured at 28 GHz when (i) only transmitting the four channels on Y-pol (single Y-pol case) and (ii) transmitting all eight channels on both X-pol and Y-pol (dual-pol case). We observe that the crosstalk deteriorates significantly when two polarizations are included (see Table 1 ), mainly because of the birefringence of the SPPs. We thus conjecture that during the machining process, some stress-induced birefringence is induced in the plates, giving rise to the observed polarization crosstalk. We also observe that the crosstalk value of channel ℓ =−1 is −23 dB at 28 GHz for the single Y-polarization case. This value increases to −19 and −20 dB when the transmitted CWs are at 27.5 and 28.5 GHz, respectively. This deterioration in crosstalk could be caused by (i) the material dispersion of our SPPs and (ii) the deviations from the design frequency of 28 GHz on the part of the SPPs. This leads to the deviation of the phase fronts of the generated OAM beams from the required azimuthal maximum variation of 2 ℓπ . Table 1 The crosstalk of OAM channels when SPPs are used for the detection. 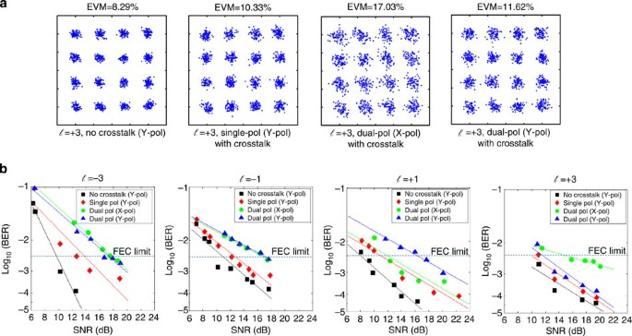Figure 4: Results of 32 Gbit s−1data transmission using eight pol-muxed mm-wave OAM channels. (a) Constellations of the received 1-Gbaud 16-QAM signals for OAM channelℓ=+3 under single Y-pol and dual-pol conditions. The SNR is 19 dB. (b) Measured BER curves of 1-Gbaud 16-QAM signals for (i) a single OAM channel (no crosstalk), (ii) four OAM channels on Y-pol (with crosstalk, Y-pol) and (iii) eight OAM channels on both X-and Y-pol (with crosstalk, X-pol and Y-pol). Full size table Figure 4a shows constellations and error vector magnitudes [27] of the received 1-Gbaud 16-QAM signals with a signal-to-noise ratio (SNR) of 19 dB for channel ℓ =+3 in both single-polarization (single-pol) and dual-polarization (dual-pol) cases. We can observe that the constellations of channels ℓ =+3 for both X-pol and Y-pol become much worse in the dual-pol case because of the fact that they experiences higher crosstalk. For similar reasons, ℓ =+3 on X-pol has a more blurred constellation than ℓ =+3 on Y-pol. The measured BERs for each channel as functions of SNR under both single Y-pol and dual-pol cases are shown in Fig. 4b . For comparison, the BER curves when only OAM channel ℓ =−1, +1, −3 or +3 is transmitted on Y-pol (in the absence of crosstalk from other channels, black square) are also shown. We see that the power penalty of each OAM channel ( ℓ =−1, +1, −3 or +3) in the single-pol case is lower than that of either polarization in the dual-pol case. This is because of the fact that each channel in the single-pol case experiences lower crosstalk than in the dual-pol case. We also observe that the OAM channel with higher crosstalk will consequently have worse BER performance, as expected. It is clear that each channel is able to achieve a raw BER below 3.8 × 10 −3 , which is a level that allows extremely low block error rates through the application of efficient forward error correction codes [28] . Neither pulse shaping nor pre-filtering technique is used at the transmitter, and the spectral efficiency in the experiment is ~16 bit s −1 Hz −1 . Expanding the potential transmission distance of an OAM channel beyond the 2.5 m achieved in our experiment depends on several factors, including the receiver aperture size (that is, size of the SPP) and the OAM beam divergence. For increased distances, less power will be received by a fixed receiver aperture due to the divergence of the OAM beam. Given that the beam diverges approximately as the square root of | ℓ |, beams with larger OAM state numbers diverge more and ultimately limit the system performance. Figure 4: Results of 32 Gbit s −1 data transmission using eight pol-muxed mm-wave OAM channels. ( a ) Constellations of the received 1-Gbaud 16-QAM signals for OAM channel ℓ =+3 under single Y-pol and dual-pol conditions. The SNR is 19 dB. ( b ) Measured BER curves of 1-Gbaud 16-QAM signals for (i) a single OAM channel (no crosstalk), (ii) four OAM channels on Y-pol (with crosstalk, Y-pol) and (iii) eight OAM channels on both X-and Y-pol (with crosstalk, X-pol and Y-pol). Full size image Separation of OAM channels using an OAM mode demultiplexer Communication systems of multiple OAM beams need to separate each data stream in order to recover any specific channel. One method that was described in the previous section used a passive power-splitting arrangement followed by individual SPPs to separate the data channels carried on each OAM state (See Fig. 2c ). In this approach, if there is an M-way power splitting, then the power loss is ( M −1)/ M and does not scale well. Similar to other types of communication systems using multiple parallel channels, it would be beneficial to the system performance to have a demultiplexer module that separates the OAM states without any added inherent power-splitting losses. In this section, we demonstrate a mm-wave OAM demultiplexer to separate multiple OAM states [29] (see Fig. 2d ). The OAM mode demultiplexer is composed of two custom-designed refractive elements that transform OAM states into transverse momentum states, which is achieved by mapping the position ( x,y ) in the input plane to a position ( u,v ) in the output plane, in which u =− a ln() and v = a tan −1 ( y / x ) (ref. 30 ). The parameter a is defined as a = d /2 π , ensuring that the transformed beam is mapped on the desired width d of the demultiplexer’s second element. The parameter b determines the position of the transformed beam along the v axis, and its value depends on the physical dimensions of the OAM mode demultiplexer. This type of mapping transforms a set of concentric rings in the input plane into a set of parallel lines in the output plane. The combination of the two refractive elements transforms the complex amplitude of the beam in the form exp ( iℓφ ), providing complex amplitude in the output plane in the form exp( iℓv / a ). A convex lens can then separate the resulting transverse momentum states into specific lateral positions, allowing for the demultiplexing of multiple states without power-splitting loss [30] , [31] , [32] . For experimental demonstrations, the refractive elements are produced from HDPE through the use of computer numerical control milling techniques. The height profile of the first element is given by [31] where L is the distance between the components. The two parameters a and b , as defined above, determine the scaling and position of the transformed beam, respectively. The height profile of the second element is given by [31] where u and v are the coordinates in the output plane. This element is placed at a distance L behind the first element. Each surface is wavelength-independent; however, dispersion effects in the material manifest themselves as defocus for different wavelengths. The system can thus be tuned to specific wavelengths by changing the distances between the elements (See Supplementary Fig. 4 and Supplementary Note 5 for more details about the OAM mode demultiplexer). To determine the spatial intensity profile after the lens of the OAM mode demultiplexer, a probe antenna is placed on a motorized 2D stage at the focal plane to measure the spatial intensity profile of the OAM beams ( ℓ =±1 and ±3) after the OAM mode demultiplexer. The intensity distribution of four different OAM beams in the desired sorting direction is measured (see Fig. 5a ), suggesting that the multiplexed OAM beams are spatially separated by the OAM mode demultiplexer. The crosstalk of the OAM channels ( ℓ =−1 and ℓ =+1) is measured to be lower than −14 dB for the single-pol case and to be lower than −12.5 dB for the dual-pol case (see Table 2 ). In this section, we transmit a 1-Gbaud QPSK signal on OAM channels with ℓ=±1 to demonstrate the mm-wave OAM mode demultiplexer. As compared with the previous section that used 16-QAM for the SPP-based receiver, we use QPSK with the demultiplexer because it currently has higher crosstalk that limits the ability to recover the higher constellation. Future improvements to the OAM demultiplexer may lead to lower crosstalk and better system performance. 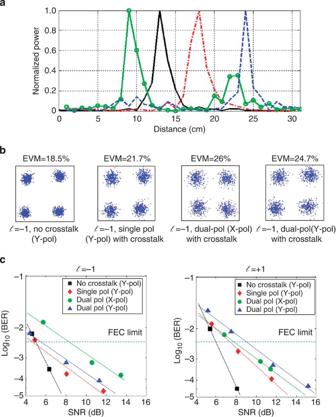Figure 5: Results of 8 Gbit s−1data transmission using mm-wave OAM mode demultiplexer for demultiplexing. (a) The normalized intensity distributions of four input OAM beams (ℓ=±1 andℓ=±3) in the OAM mode sorting direction in the detection plane. (b) The received constellations of the 1-Gbaud QPSK signals for OAM channelℓ=−1 in single Y-pol and dual-pol cases with an SNR=11 dB. (c) Measured BER curves of 1-Gbaud QPSK signals for (i) a single OAM channel (no crosstalk), (ii) two OAM channels on Y-pol (with crosstalk, Y-pol) and (iii) four OAM channels on both X-and Y-pol (with crosstalk, X-pol and Y-pol). Figure 5b shows the constellations and error vector magnitudes of the received 1-Gbaud QPSK signals with an SNR of 11 dB for channel ℓ =−1 in both single- and dual-polarization cases. The BERs of the OAM channels ℓ =−1 and ℓ =+1 are depicted as functions of SNR in Fig. 5c . We see that each OAM channel in the single-pol case, for which the crosstalk is lower, has a lower power penalty than that of either polarization in the dual-pol case. We also observe that each OAM channel can achieve a raw BER below the forward error correction limit of 3.8 × 10 −3 . Figure 5: Results of 8 Gbit s −1 data transmission using mm-wave OAM mode demultiplexer for demultiplexing. ( a ) The normalized intensity distributions of four input OAM beams ( ℓ =±1 and ℓ =±3) in the OAM mode sorting direction in the detection plane. ( b ) The received constellations of the 1-Gbaud QPSK signals for OAM channel ℓ =−1 in single Y-pol and dual-pol cases with an SNR=11 dB. ( c ) Measured BER curves of 1-Gbaud QPSK signals for (i) a single OAM channel (no crosstalk), (ii) two OAM channels on Y-pol (with crosstalk, Y-pol) and (iii) four OAM channels on both X-and Y-pol (with crosstalk, X-pol and Y-pol). Full size image Table 2 The crosstalk of OAM channels when the mm-wave mode demultiplexer is used for detection. Full size table Our experiment takes place in the near-field because the distance is shorter than the Fraunhofer distance [23] . We believe this approach could potentially be expanded to longer distances in the far field [18] , as long as sufficient power and phase change of each OAM beam is captured. Moreover, atmospheric turbulence would likely not present a critical challenge for this frequency range [33] . In general, the number of OAM beams that can be accommodated in a system is limited by different factors, including receiver aperture size and intermodal crosstalk. Given a fixed receiver aperture size, a larger OAM ℓ value may result in a larger beam size at the receiver such that the recovered power decreases and the BER increases. In addition, higher intermodal crosstalk leads to an increase in power penalty and a limited number of available OAM states. Intermodal crosstalk can arise because of many factors, including imperfect components [4] , system misalignment [22] and the effects of the transmission medium [33] . An OAM-based communication system faces several challenges as to its ability to scale to higher numbers of OAM beams. Issues include reducing intermodal crosstalk, improving the demultiplexer and developing integrated devices. We emphasize that our implementation of OAM multiplexing is different from traditional RF spatial multiplexing [34] , [35] , [36] . The latter employs multiple spatially separated transmitter and receiver aperture pairs for the transmission of multiple data streams. As each of the antenna elements receives a different superposition of the different transmitted signals, each of the original channels can be demultiplexed through the use of electronic digital signal processing. In our implementation, the multiplexed beams are completely coaxial throughout the transmission medium and use only one transmitter and receiver aperture (although with certain minimum aperture sizes), employing OAM beam orthogonality to achieve efficient demultiplexing without the need for further digital signal post-processing to cancel channel interference [23] . There are thus significant implementation differences between the two approaches (for further discussions on the fundamental relationship between conventional spatial multiplexing and OAM multiplexing, we refer the reader to refs 37 , 38 , 39 ). Generation and multiplexing of OAM channels Each of the OAM-carrying mm-waves on two orthogonal polarizations is generated with a specifically designed SPP, which introduces a helical phase front to the data-carrying Gaussian beam. The vortex charge of the OAM beam is determined by the phase variations along the azimuthal angle. Eight OAM beams are coaxially multiplexed via cascaded 50:50 mm-wave BSs that are designed to operate at a frequency of 28 GHz. The OAM-carrying EM waves maintain orthogonality while propagating coaxially in free space. Detection of OAM channels We recover the data channels carried by a specific OAM state ℓ by passing all the beams of different OAM states through an SPP. This SPP has an inverse value of − ℓ with regard to the data we wish to recover. Using this approach, only the desired OAM beams will be converted into Gaussian-like beams ( ℓ =0) and be efficiently coupled into the receiver antenna. Alternatively, multiple coaxially propagating OAM beams can be separated by using an OAM mode demultiplexer, which performs a log-polar geometrical transformation and unfolds the vortex beams into tilted plane waves. A convex lens can then focus each tilted plane wave at a specific position in the focal plane, which corresponds to a specific receiver aperture, and thus enable the detection of multiple OAM channels without power-splitting loss. How to cite this article: Yan, Y. et al. High-capacity millimetre-wave communications with orbital angular momentum multiplexing. Nat. Commun. 5:4876 doi: 10.1038/ncomms5876 (2014).